Genome-wide association study identifies variants at 16p13 associated with survival in multiple myeloma patients Here we perform the first genome-wide association study (GWAS) of multiple myeloma (MM) survival. In a meta-analysis of 306 MM patients treated at UCSF and 239 patients treated at the Mayo clinic, we find a significant association between SNPs near the gene FOPNL on chromosome 16p13 and survival (rs72773978; P =6 × 10 −10 ). Patients with the minor allele are at increased risk for mortality (HR: 2.65; 95% CI: 1.94–3.58) relative to patients homozygous for the major allele. We replicate the association in the IMMEnSE cohort including 772 patients, and a University of Utah cohort including 318 patients (rs72773978 P =0.044). Using publicly available data, we find that the minor allele was associated with increased expression of FOPNL and increased expression of FOPNL was associated with higher expression of centrosomal genes and with shorter survival. Polymorphisms at the FOPNL locus are associated with survival among MM patients. Multiple myeloma (MM) is an incurable haematological malignancy of plasma cells. Approximately 22,000 new cases are diagnosed each year in the United States and over 10,000 deaths occur annually [1] . Family history is a strong risk factor for MM [2] . Recent genome-wide association studies (GWAS) reported eight loci associated with susceptibility to MM [3] , [4] , [5] . A variety of clinical features and biomarkers are associated with MM prognosis [6] . Chromosomal abnormalities are also associated with prognosis; deletions at 17p, 13q, amplifications at 1q and translocations t(4;14) and t(14;16) have been associated with a poor prognosis, while hyperdiploidy is associated with a favourable prognosis [7] , [8] , [9] . Gene expression signatures of the myeloma cells also predict survival [10] , [11] , [12] , [13] , [14] . Germline genetic variants are associated with survival among patients with oesophageal [15] , breast [16] , [17] , pancreatic [18] , [19] and small cell lung cancer [20] . We performed the first GWAS of MM survival, by conducting a meta-analysis of two studies from the University of California San Francisco (UCSF) and the Mayo Clinic. We found a locus on chromosome 16 associated with survival. We replicated the findings in the International Multiple Myeloma rESEarch (IMMEnSE) consortium and the University of Utah cohort. The top single-nucleotide polymorphisms (SNPs) were at the FOPNL locus. Using publicly available data of gene expression from peripheral blood of normal individuals, we found that the risk alleles at the top SNPs were associated with increased expression of FOPNL . We also found that increased expression of FOPNL was associated with higher ‘centrosome index’, a gene expression correlate of centrosome amplification in MM cells, which has been associated with poor survival. 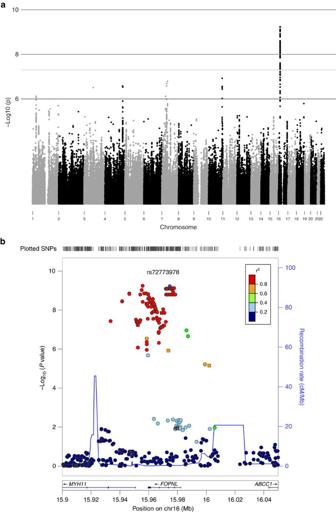Figure 1: GWAS results for survival among MM patients. (a) Manhattan plot of results of genome-wide association analysis for survival in MM patients. Each point represents the negative logPvalue of the meta-analysis for association with survival using the UCSF and Mayo Clinic data. (b) Locuszoom plot for association statistics at the 16p13 region in the meta-analysis of UCSF and Mayo. Each dot represents the negative logPvalue for the association statistics from the meta-analysis. The top associated SNP (rs72773978) is coloured in purple and the remaining SNPs are coloured according to linkage disequilibrium values (r2) with the top SNP. Identifying a locus for survival We performed a GWAS of overall survival among MM patients in cohorts ( Table 1 ) from UCSF ( n =306) and Mayo Clinic ( n =239) separately. One locus mapping to chromosome 16p13.11 (Hg19) showed a suggestive association in both the UCSF ( P =8.4 × 10 –7 ; proportional hazards model) and the Mayo Clinic studies ( P =1.1 × 10 –4 ; proportional hazards model). In a meta-analysis of these GWAS, the locus was genome-wide significant ( Fig. 1a ) with the strongest evidence at two SNPs in perfect linkage disequilibrium rs72773978 and rs117863986 ( P =6.0 × 10 –10 for both; meta-analysis P value is calculated using inverse variance-based weighting). We found no significant deviation from the proportional hazards assumption for the top SNP in either the UCSF ( P =0.74; P values calculated by testing whether scaled Schoenfeld residuals vary with time) or Mayo clinic studies ( P =0.95). We identified 131 SNPs at this locus associated with survival at P <5x10 –8 ( Supplementary Data 1 ); these SNPs had ∼ 5–7% minor allele frequency (MAF) and were in tight linkage disequilibrium ( r 2 >0.8) with the top SNPs ( Fig. 1b ). Of the 131 top SNPs, 17 were genotyped in the UCSF data set and 1 was genotyped in the Mayo Clinic data set ( Supplementary Data 1 ). The remaining SNPs were imputed but had very high imputation quality scores (Information >0.9 or r 2 >0.9). We directly genotyped eight additional SNPs in the Mayo clinic data set, including one of the top two SNPs, rs117863986, and found consistently strong levels of association with the genotyped SNPs (rs117863986 hazard ratio (HR): 2.26; 95% confidence interval (CI): 1.46–3.40; P =0.00021; proportional hazards model) and other SNPs ( Supplementary Table 1 ). Table 1 Clinical characteristics of patients in discovery and replication studies. Full size table Figure 1: GWAS results for survival among MM patients. ( a ) Manhattan plot of results of genome-wide association analysis for survival in MM patients. Each point represents the negative log P value of the meta-analysis for association with survival using the UCSF and Mayo Clinic data. ( b ) Locuszoom plot for association statistics at the 16p13 region in the meta-analysis of UCSF and Mayo. Each dot represents the negative log P value for the association statistics from the meta-analysis. The top associated SNP (rs72773978) is coloured in purple and the remaining SNPs are coloured according to linkage disequilibrium values ( r 2 ) with the top SNP. Full size image Analysis of the genome-wide distribution of association statistics ( Supplementary Fig. 1a ) revealed minimal deviation from the expectation under the null (lambda=1.002). After removing SNPs from a 200-kB region around the top locus on chromosome 16, we found no evidence for additional signal genome wide ( Supplementary Fig. 1b ), although some other loci had some suggestive signals with P values 5 × 10 –7 –1 × 10 –7 ( Supplementary Data 1 ). The UCSF study had a median time of 7.6 months (interquartile range 5.7–8.9 months) between the date of diagnosis and the date of ascertainment. Therefore, we considered whether this delay affected our results. 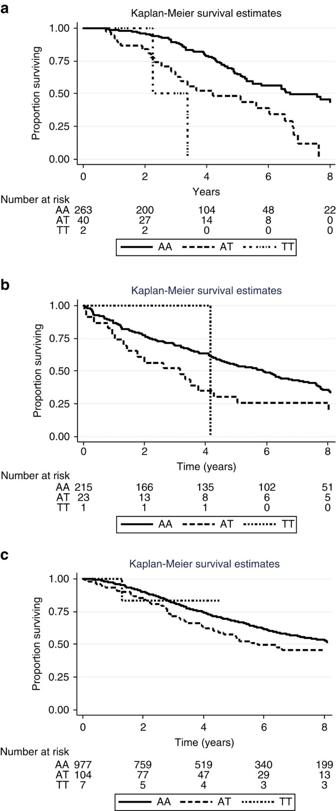Figure 2: Kaplan–Meier Survivorship plot by genotype for rs72773978. (a) UCSF (N=306); (b) Mayo (N=239) and (c) IMMENSE/Utah (N=1,080) studies. We plotted the results by genotype. To generate the plots for the discovery data sets, we rounded the imputation results to the nearest whole numbers to infer genotypes of individuals. First, we adjusted for the time difference between the date of diagnosis and ascertainment in the proportional hazards models and found no attenuation ( Supplementary Table 2 ). We also considered models stratified by the delay between date of diagnosis and ascertainment ( Supplementary Table 2 ). We found that the effect was consistent among patients enrolled between 0 and 5.9 months after diagnosis (HR: 3.23; 95% CI: 1.28–8.17; P =0.013; proportional hazards model) those enrolled between 6 and 11.9 months after diagnosis (HR: 3.04; 95% CI: 1.67–5.55; P =0.00028; proportional hazards model) and those enrolled from 12 to 23.9 months (HR: 5.06; 95% CI: 1.18–21.79; P =0.029; proportional hazards model). Thus, we concluded that the delay between diagnosis and ascertainment within the first 2 years was unlikely to affect the association between the SNP and overall survival. We also considered models that adjusted for the difference between date of diagnosis and ascertainment in the Mayo study and found no change in the association as expected ( Supplementary Table 2 ), since nearly all of the participants were ascertained within 1 month of diagnosis. We searched for additional SNPs that were associated independently of the top SNP by performing conditional analyses including rs72773978 and other SNPs within 100 kB of that SNP. We performed survival analyses for all SNPs that were either in no lethal dose (LD; R 2 <0.1) or in modest LD ( R 2 0.1–0.5) with RS72773978, adjusting for the effect of principal components (PC’s) and for the effect of RS72773978. We found no other significant associations in the locus after adjusting for multiple hypothesis testing. The median survival was decreased by ∼ 2.7 years among patients who were either heterozygous or homozygous for the rare variant (T allele) of rs72773978 compared with patients homozygous for the common variant in both the UCSF and Mayo Clinic cohorts ( Fig. 2 ). In models that adjusted for age, gender and genetic ancestry, ∼ 10–14% of patients had an increased risk of death (hazard ratio ∼ 2.6; Table 2 ) in the meta-analysis of these two data sets. Figure 2: Kaplan–Meier Survivorship plot by genotype for rs72773978. ( a ) UCSF ( N =306); ( b ) Mayo ( N =239) and ( c ) IMMENSE/Utah ( N =1,080) studies. We plotted the results by genotype. To generate the plots for the discovery data sets, we rounded the imputation results to the nearest whole numbers to infer genotypes of individuals. Full size image Table 2 Association of rs72773978 and MM survival. Full size table We also performed a separate analysis of individuals who genetically clustered with Caucasians in the UCSF data set ( Supplementary Fig. 2 ). We repeated the meta-analysis of the Mayo Clinic data with the UCSF Caucasian-only sample ( Supplementary Table 3 ), and found that the association with rs72773978 remained significant ( P =2.4 × 10 –9 ; proportional hazards model). The UCSF cohort included African American patients ( N =25) and patients of Latino ( N =27) or other patients who clustered with those of mixed ancestry ( N =24). In an analysis of these patients, we also found a nominally significant association between shorter survival and the minor allele (HR: 2.43; 95% CI: 1.09–5.39; P =0.029 proportional hazards model). We also examined whether the top SNPs that we identified were associated with susceptibility to MM in our two studies. We found no significant difference in genotype frequencies between cases and controls ( Supplementary Table 4 ). Relationship to stage at diagnosis and treatment We evaluated the effect of the genotype on survival after adjustment for the clinical stage. In analyses that adjusted for stage using either the international staging system (ISS) definition or the Durie–Salmon staging system, the rs72773978 genotype remained a strong predictor of survival ( Table 2 ). Among the participants in the Mayo Clinic on whom LDH levels were available ( N =154), we saw a consistent level of association (HR: 2.25; 95% CI: 1.26–4.03; P =0.006; proportional hazards model). Since MM treatment has improved significantly in the last decade, we used data available from both cohorts to determine whether the SNP effect varied by initial treatment ( Supplementary Table 5 ). We found a consistent effect of the SNP regardless of the type of treatment initiated ( Table 3 ) and no evidence of interaction between treatment and the SNP in either the UCSF ( P =0.9; P for interaction derived using proportional hazards model) or Mayo Clinic ( P =0.52; P for interaction derived using proportional hazards model) cohorts. Table 3 Effect of SNP by initial treatment among patients in the UCSF cohort. Full size table Among patients in the Mayo Clinic study, 134 (56%) were treated with both high-dose chemotherapy (HDC) followed by autologous stem cell rescue. We adjusted for HDC in the proportional hazards models and found that, although HDC was a strong predictor of longer survival in the cohort, there was only mild attenuation of the SNP association with survival ( Supplementary Table 6 ). Since nearly all (97%) of the UCSF patients received HDC, the same analysis could not be performed within the UCSF study. Replication We replicated the association of top SNPs from the UCSF and Mayo Clinic meta-analysis in a replication meta-analysis of 1,090 MM cases, including 772 European MM patients from the IMMEnSE consortium and 318 from the Utah cohort ( Supplementary Table 7 ). We selected two SNPs for replication including rs72773978, one of the top associated SNPs from the meta-analysis and rs12598966, a SNP resulting in an amino-acid substitution in the FOPNL gene. We performed a meta-analysis of all of the replication studies and found a significant association between rs72773978 and survival in the replication cohorts adjusted by age and sex (HR: 1.34; 95% CI: 1.01–1.74; P =0.044; proportional hazards model) with survival shorter by ∼ 1.2 years among carriers of the minor allele ( Fig. 2c ). There was no evidence of heterogeneity of effect within the replication studies ( P =0.14; χ 2 -test for heterogeneity). The other SNP, rs12598966, was not significantly associated with survival in the replication. We noted a slightly stronger effect size in analyses that adjusted for stage. However, the change in effect size was not due to negative confounding between stage and the SNP, but rather to the fact that the cohorts with missing data on stage were the ones with an inconsistent point estimate ( Supplementary Table 3 ). In a meta-analysis that did not adjust for the ISS stage but just included participants without missing data on the ISS stage, we saw approximately the same effect size (HR: 1.71; 95% CI: 1.18–2.47; P =0.005; proportional hazards model) as in the meta-analysis that adjusted for the ISS stage ( Supplementary Table 7 ). Analysis of function The top SNPs were in a region that overlapped the entire FOPNL gene and a portion of the MYH11 gene ( Fig. 1b ). In addition, known drug transporters, ABCC1 and ABCC6 , are located ∼ 50 and 300 kb away, respectively. One of the top SNPs, rs12598966, is located in the coding sequence of FOPNL and leads to a nonsynonymous amino-acid substitution: Glu->Lys at amino acid 156; however, this SNP was not significantly associated with survival in the replication and was not predicted to have a deleterious effect on protein function (sorting intolerant from tolerant (SIFT) score=0.89 and Polyphen 2 score=0.275). Next, we investigated the top 145 SNPs (all in tight LD ( r 2 >0.8) with rs72773978) for an effect on gene expression using GENEVAR [21] . The top two SNPs, rs72773978 and rs117863986, were not included in the database; however, six other SNPs in strong LD ( r 2 =1) with rs72773978 are present in the database and are associated with expression of FOPNL ( Supplementary Table 8 ). The minor allele of these SNPs predicted higher expression of FOPNL. There was no significant association between these SNPs and expression of other genes within 1 MB of the locus. We identified 13 SNPs in LD with rs72773978 as being potentially functional ( Supplementary Table 9 ). Six of these SNPs are in the 3′ untranslated repeat of the FOPNL gene and, therefore, may be involved in transcript stability. Seven SNPs were identified as being in sites of open chromatin and thus may be involved in transcriptional regulation. Since the top SNPs were associated with gene expression, we hypothesized that expression of FOPNL may be associated with survival among MM patients. In particular, higher expression of FOPNL is associated with the minor allele of the top SNPs from the GWAS and should also be associated with shorter survival. We used publicly available data on gene expression (GSE2658) and survival from 414 MM cases to test this hypothesis [13] . As predicted, we found a significant association between higher expression of FOPNL and worse survival ( Supplementary Table 10 ). FOPNL is known to localize to the centrosome and the pericentriolar satellites. Since centrosome amplification is known to be a predictor of poor prognosis, we evaluated the association between FOPNL expression and the centrosome index, a previously validated gene expression signature of centrosome amplification. We found a very strong correlation ( Supplementary Table 11 ) between higher FOPNL expression and increased centrosome index in the study we analysed for survival (GSE2658) and in two additional studies (GSE19784 and GSE26760). We performed a GWAS for survival among MM patients and identified SNPs at chromosome 16p13 that were strongly associated with mortality. The SNPs were in the region of the FOPNL gene and a subset of the SNPs were associated with FOPNL expression levels, with the minor allele predicting higher expression [22] . We also found that FOPNL expression was associated with poorer survival using data from a previous study [13] . Thus, our results strongly suggest that FOPNL is a gene involved in myeloma progression. FOPNL is known to be associated with centrosome function [23] , [24] . Centrosome amplification is common in MM and is associated with poor prognosis [25] , [26] . Furthermore, inhibition of centrosomal clustering may be effective in treatment of MM [27] , [28] . We found that germline variation that affects a gene involved in centrosomal function may also contribute to disease progression. Furthermore, we found an association between FOPNL expression and centrosome index in three data sets of gene expression from myeloma samples. However, our results implicating FOPNL as the causal gene at this locus rely on the synthesis of several data sets. We were not able to directly correlate the SNPs with gene expression, centrosome index and survival in the same data set. It is possible that another gene/s at this locus may be responsible for the effect we observe, or that the effect is mediated by FOPNL, but that it is not through a mechanism related to centrosome amplification. Additional studies of this gene and centrosomal function will help to further define the mechanism underlying the association that we identified. Our results imply that germline genetic variation is associated with survival among patients with MM. Other GWAS have identified loci that affect survival in other cancer types [15] , [16] , [17] , [18] , [20] . At least one of the known loci for MM susceptibility is associated with the risk for a particular subtype of MM [4] , which may also have an effect on prognosis. MM is a heterogeneous disease with substantial variation in prognosis among different patients. Identifying patients who are at higher risk of progression may be of importance in treating these patients more aggressively earlier in their disease. Our results identify the FOPNL genotype as a predictor of survival, and we found that the association remains significant after adjustment for stage at diagnosis. However, the effect size we observed in the replication cohorts was substantially attenuated compared with the effect size in the discovery cohorts. This difference is most likely because of ‘winner’s curse’—a tendency for the initial study to overestimate the true effect size [29] . Thus, the replication cohorts in our study are more likely to represent the true effect size in future studies. Our study has several important limitations. We could not examine the association between SNPs and MM survival by cytogenetic abnormalities since the majority of our patients were diagnosed before the common use of cytogenetic and fluorescent in situ hybridization analyses in clinical practice. Therefore, it will be important to examine the utility of this genotype in the setting of cytogenetic and fluorescent in situ hybridization analyses and gene expression signatures. Furthermore, we could not adjust for gene expression patterns, which are also known to be associated with survival. We found no difference between patients who were initially treated with modern versus older therapies. However, our ability to analyse the SNP using different therapies was limited to the UCSF data set and we had inadequate power to detect interactions between the SNPs and particular drugs. Furthermore, we only adjusted for the association between initial treatment and survival, and it is likely that many of the patients who were initially treated with older regimens received newer regimens if they survived to the era when these became available. It is possible that the effect that we saw is modified by one regimen or by one class of medications. Additional studies should be conducted in the context of clinical trials or other cohorts where treatment regimens are more uniform to investigate whether the effect of the locus we identified is modified by particular treatments. In summary, we found a strong association between a locus on chromosome 16p and MM survival that is likely due to an effect on expression of the FOPNL gene. The SNPs we identified may become important clinical predictors of outcome among MM patients. Participants UCSF study : The UCSF Institutional Review Board (IRB) approved ascertainment of cases and use of existing biospecimens for genetic analysis. All participants gave informed consent. The study included 370 patients treated for MM at UCSF between 1989 and 2010. We excluded 10 samples because of insufficient clinical data. We also excluded 42 participants whose blood was collected ≥2 years after diagnosis from the survival analysis because of the potential bias towards long-term survivors among these participants. The median delay between diagnosis and ascertainment among the 42 participants excluded was 2.9 years (interquartile range 2.4–4.7 years). The median delay among the participants included was 7.6 months (interquartile range 5.7–8.9 months). We used white blood cells harvested after mobilization of stem cells with granulocyte colony-stimulating factor as a source of DNA. Mobilization of stem cells is performed before HDC followed by autologous stem cell transplantation. The patient receives granulocyte colony-stimulating factor and then undergoes harvesting of peripheral white blood cells via apheresis several days later [30] , [31] . Bone marrow stem cell fraction is monitored via CD34 antibody, and apheresis is continued until an adequate number of CD34+ cells have been collected for stem cell rescue. The cells are then stored in liquid nitrogen. We ascertained the date of death using chart reviews and death registry data. Survival time was determined as the date of diagnosis until date of death or last clinic visit for patients who were not known to have died. Clinical stage and initial chemotherapy regimen was determined by chart review. For analysis of treatment, we dichotomized treatments into either newer regimens (including an Imid and/or proteasome inhibitor) or older regimens (including neither an Imid nor proteasome inhibitor). Nearly all of the participants in the UCSF study (>97%) received HDC with stem cell rescue (autologous bone marrow transplant). Mayo Clinic study : Ascertainment of MM cases and genotyping was approved by the Mayo Clinic IRB. The study included incident MM cases seen in the regional practice between 1998 and 2007 and recruited within 6 months of initial diagnosis. Nearly all participants (96%) were recruited within 1 month of diagnosis and, the remainder were recruited between 1 and 5.5 months after diagnosis. Eligible cases provided consent and a blood sample for research studies of MM. A total of 243 MM cases were used for analyses. DNA was extracted from stored peripheral blood samples. We ascertained date of death and calculated survival time as described for the UCSF study. The clinical stage was determined by chart review. Clinical data on survival could be ascertained on 239 patients. Initial chemotherapy regimen and use of HDC was determined by chart review. For analysis of treatment, we dichotomized treatments into either newer regimens (including an Imid and/or proteasome inhibitor) or older regimens (including neither an Imid nor proteasome Inhibitor). Approximately 56% of participants were treated with autologous stem cell transplant. IMMEnSE study : The IMMEnSE consortium is a case–control study recruited from seven different European and North American countries [32] . MM cases are defined by a confirmed diagnosis of MM, according to the International Myeloma Working Group criteria [33] . For each patient, demographic and clinical parameters at diagnosis and survival were collected by the responsible clinicians in each of the IMMEnSE centres. The data collected are standardized in a central database kept at the German Cancer Research Center (DKFZ, Heidelberg, Germany). For each subject, a sample of peripheral blood or extracted DNA has been collected and sent to DKFZ. A total of 772 MM cases with survival information available in the IMMEnSE consortium were included in this study. Utah study : Sampling and genetic analysis was approved by the University of Utah IRB. The study included prevalent MM cases in the state of Utah, ascertained up to 2012. Eligible cases provided consent and a blood or saliva sample from which DNA was extracted. Date of diagnosis was confirmed from chart review and Utah Cancer Registry data. Date of death was confirmed from chart review and death registry data. Survival time was determined as the date of diagnosis until the date of death, last contact with the study or last known event in Utah (determined from statewide vital records, driver’s license renewals and voter registrations in the Utah Population Database) for patients who were not known to have died. A total of 318 MM cases with DNA and survival information were available for this study. GWAS genotyping and imputation All SNP positions were annotated using the Genome Reference Consortium GRCh37 (Hg19) version of the human genome. UCSF : A pilot study of 81 MM samples used an Illumina 660 array genotyped at the UCSF Genomics Core Facility. In a second phase, we genotyped 289 MM samples using an Illumina Omni5 array at Expression Analysis (Durham, NC). Of the 370 participants in the GWAS, 52 participants were excluded from the survival analysis as noted above because of either insufficient clinical data ( N =10) or because of >2 year time difference between diagnosis and ascertainment ( N =42). Of the remaining 318 samples we dropped 12 since they did not pass quality control for genotyping. Eleven were dropped because of high missing genotype values (>5% missing genotypes per sample) and one sample was dropped because of potential contamination, leaving 306 patients. We dropped SNPs that had >5% missing values or were monomorphic. Imputation was performed using IMPUTE2 (ref. 34 ; https://mathgen.stats.ox.ac.uk/impute/impute_v2.html#home ) with all samples from 1000 Genomes data set (Version 2, May 2011 release [35] ) as a reference. Imputed SNPs with Information<0.5 or MAF<0.025 were excluded, leaving 8,036,255 SNPs for analysis. Mayo Clinic: Cases were genotyped using the Affymetrix 6.0 array. Monomorphic SNPs and those with a call rate <95% were excluded, leaving 786,950 observed SNPs. Four samples with call rates <95% and one sample with non-European ancestry according to principal components analysis were excluded, leaving 243 MM cases and 239 with follow-up past date of diagnosis. Imputation was performed with BEAGLE [36] ( http://faculty.washington.edu/browning/beagle/beagle.html ), using all samples from version 2 of the 1,000 Genomes data (May 2011 release) as reference. Imputed SNPs with an r 2 <0.3 or MAF<0.025 were excluded, leaving 7,276,170 SNPs for further analyses. Replication genotyping We selected two SNPs for replication in IMMEnSE and Utah samples including one of the top two SNPs from the meta-analysis (rs72773978) and a SNP in high linkage disequilibrium with the top SNP, encoding a nonsynonymous amino-acid substitution in FOPNL (rs12598966). These SNPs were typed using 5′ exonuclease (TaqMan) assays (ABI) at the German Cancer Research Center (DKFZ) in Heidelberg (IMMEnSE samples) and at the Genomics Core at the University of Utah (Utah samples). Duplicates of 12% of the samples were interspersed throughout the plates and concordance rate among duplicates was >99.9%. Statistical analysis We performed genome-wide analyses for association with survival using proportional hazards models in the UCSF and Mayo data sets separately. We inferred genetic ancestry using principal components analysis (PCA) in each cohort using SmartPCA [37] . Each SNP was entered into the model under an assumption of log-additive increased risk, and adjusting for PC’s 1–3, age and gender. Imputed SNPs were modelled using the probability of genotypes. We tested the proportional hazards assumption for the top SNPs by calculating the scaled Schoenfeld residuals and testing whether they are significantly associated with time [38] . We also performed a subset analysis of Caucasians only in the UCSF data set. We identified Caucasians on the basis of genetic ancestry (see Supplementary Fig. 2 ). Individuals who clustered with self-described Caucasians (PC1>0, PC2<0) were included in this subset analysis ( N =229). All analyses were performed in R. For graphing survival results, we used the Kaplan–Meier estimates of the survival function and graphed the results using Stata (Version 10). We graphed the association statistics for all SNPs near the top locus using LocusZoom [39] . We used Cox regression models adjusted for age and gender to test the association between SNPs and survival in the IMMEnSE consortium and the Utah cohort. We performed a meta-analysis of the UCSF and Mayo Clinic results on a total of 6,026,834 SNPs in common from both GWAS that met the allele frequency and imputation quality thresholds. We also conducted a meta-analysis of data on two top SNPs from seven centres within the IMMEnSE consortium and the Utah study in our replication study. We calculated a fixed effects model for each SNP using METAL [40] . We used Cochran's Q statistic to test for heterogeneity. To examine the association of SNPs and risk of MM, we compared the genotype frequencies of cases versus ethnically matched controls from the UCSF ( N =298) and the Mayo Clinic ( N =295) sites, respectively. We used logistic regression models, adjusting for PC1–3 age and gender. Expression quantitative trait locus (eQTL) analysis We used the data set from ref. 22 for eQTL analyses, which consists of 856 Caucasian individuals including 154 monozygotic twin pairs, 232 dizygotic twin pairs and 84 singletons. We focused on expression in lymphocytes in this data set. We used GENEVAR [21] to query the top 145 SNPs from the GWAS and identified 6 SNPs, that were also in the data set described in ref. 22 . We queried GENEVAR for beta coefficients and P values for associations between six SNPs and the genes within a 1-Mb window, including FOPNL, MYH11, ABCC1, NDE1, KIAA0430, ABCC6, RRN3, NTAN1 KIAA0250 and KIAA0251 . Gene expression and centrosome index We downloaded gene expression data from refs 13 , 41 , 42 from the National Institutes of Health Gene Expression Omnibus (accession number: GSE2658, GSE19784 and GSE26760, respectively). [13] consisted of gene expression data from 559 MM samples assayed on Affymetrix U133 arrays; ref. 41 consisted of gene expression data from purified CD138+ plasma cells of 320 newly diagnosed myeloma patients using Affymetrix GeneChip U133 plus 2.0 arrays; ref. 42 consisted of 304 CD138-purified bone marrow samples from patients with MM were analysed on Affymetrix U133 Plus 2.0 microarrays. Gene expression and MM outcome : Of the samples in the Zhan et al. [13] data set, 414 also had available clinical data and were included in the original publication and, therefore, we used the data from these 414 samples in our analyses. We used log-transformed probe intensity values as predictors of survival, entering these as continuous variables into a proportional hazards model. We analysed each of the two probes for FOPNL on the Affymetrix U133 array separately and also considered the average of the two probes as a predictor of overall survival in the proportional hazards model. Analysis of potential SNP function : We used SIFT [43] and Polyphen2 (ref. 44 ) to determine the likelihood that a nonsynonymous amino-acid substitution has a deleterious effect on protein function. We used FunciSNP [45] to determine whether any of the SNPs may affect gene expression, including any SNPs with R 2 >0.7 with rs72773928. R 2 values for linkage disequilibrium were calculated in European ancestry samples from 1,000 genomes. How to cite this article : Ziv, E. et al. Genome-wide association study identifies variants at 16p13 associated with survival in multiple myeloma patients. Nat. Commun. 6:7539 doi: 10.1038/ncomms8539 (2015).